Local endocytosis triggers dendritic thinning and pruning inDrosophilasensory neurons The refinement of neural circuits involves dendrite pruning, a process that removes inappropriate projections that are formed during development. In Drosophila sensory neurons, compartmentalized calcium (Ca 2+ ) transients in dendrites act as spatiotemporal cues to trigger pruning, yet how neurons define the dendrites with Ca 2+ transients remains elusive. Here we report that local elevation of endocytic activity contributes to defining dendrites that generate Ca 2+ transients, triggering pruning. In vivo imaging of single dendrites reveals an increase of endocytosis in proximal dendrites that spatially and temporally correlates with dendrite thinning, an early step in pruning tightly coupled with compartmentalized Ca 2+ transients. Two GTPases, Rab5 and dynamin, are required for both the increased endocytic activity and compartmentalized Ca 2+ transients. Further genetic analyses suggest that local endocytosis in proximal dendrites functions cooperatively with global endocytosis-mediated protein degradation pathways to promote dendrite pruning. In the developing brain of vertebrates and invertebrates, after axon/dendrite outgrowth and synapse formation, neurons prune their axons and dendrites to eliminate excessive or inappropriate connections that initially formed during early development [1] , [2] . For example, layer V neurons in the visual cortex of rats degenerate the distal compartment of the primary axons that is initially formed during early development and extends to the spinal cord [3] . Likewise, mitral and tufted cells in the olfactory bulb of rats initially have multiple primary dendrites that contact adjacent glomeruli; however, they eventually lose all but one dendritic branch that remains in contact with a single glomerulus [4] . In the refinement processes, a substantial portion of neuronal branches is often eliminated by local degeneration, in which a group of neuronal branches distal from a boundary point in a neuron is degenerated simultaneously [2] , [5] . Such large-scale pruning is thus achieved in a compartmentalized manner within the entire neuronal processes. Therefore, proper pruning critically depends on local activation of the machinery at the boundary that defines the branches to be or not to be degenerated. Drosophila dendrite arborization sensory neurons are an excellent model for studying developmental dendrite pruning because dendritic branches can be visualized by live imaging during the entire pruning process, and these neurons are amenable to genetic manipulations including overexpression and/or downregulation of genes of interest in vivo [6] , [7] , [8] . This is most strikingly exemplified by class IV dendrite arborization (C4da) sensory neurons that undergo dendrite pruning during early metamorphosis [9] , [10] , [11] . Pruning of C4da dendrites follows a stereotyped chain of events: dendrites become thinner and are subsequently severed at the proximal regions by ~5 h after puparium formation (a.p.f. ), after which distal portions of the dendrite arbor degenerate within several hours [11] , [12] , [13] . Thus, dendrite pruning of C4da neurons occurs in a compartmentalization- and degeneration-based manner. Caspases are required for the distal degeneration of severed dendrites [14] and possibly also in the proximal severing [15] , [16] . Although recent genetic studies have identified additional components of the machinery involved in remodelling the dendritic cytoskeleton, severing dendrites and the clearance of pruned dendrites [10] , [17] , [18] , little is known about spatial regulation of the process. Although the cellular and molecular mechanisms that act locally to define dendritic branches destined to be pruned are largely unknown, recent findings indicate that localized Ca 2+ signalling regulates dendrite pruning of Drosophila C4da neurons [19] . Spontaneous Ca 2+ transients commence in a compartmentalized manner in groups of C4da dendrites before pruning in early metamorphosis, and dendrites are eventually pruned away in the temporal order in which they experience the Ca 2+ transients, in part through the activation of the Ca 2+ -dependent protease calpains. These data demonstrate that the compartmentalized Ca 2+ transients provide spatial and temporal information about dendrite pruning. These Ca 2+ transients mostly emerge in distal dendrites with obvious boundary points between branches with and without Ca 2+ transients. Once Ca 2+ transients commence in a particular group of dendritic branches, the transients continue to occur in the same regions with the same boundary points. Thus, the boundary points that compartmentalize the dendritic Ca 2+ transients appear to be established at the proximal branches ~3 h before the dendrite degeneration. In this study, by taking advantage of the compartmentalized Ca 2+ transients in Drosophila C4da dendrites, which allows us to visualize the dendritic branches destined to be pruned ~3 h before the branch removal, we characterize the cellular and molecular mechanisms that compartmentalize the Ca 2+ transients in particular dendritic branches. Among the cellular events that are observed in the proximal dendrites at the time when Ca 2+ transients commenced, dendrite thinning at the proximal branches correlates spatially and temporally with appearance of the dendritic Ca 2+ transients. By performing high-resolution live imaging experiments, we demonstrate that endocytic activity is locally and transiently elevated at the proximal branches, where dendrites underwent thinning. We further identify the two GTPases Rab5 and dynamin as the critical factors for the elevated endocytic activity in the proximal dendrites. Genetic inhibition of these two GTPases in C4da neurons causes complete loss of dendrite thinning in proximal dendrites. Under this condition, both Ca 2+ transients and dendrite pruning are impaired. These data suggest an intriguing possibility that the local endocytosis-mediated dendrite thinning defines dendrites with compartmentalized Ca 2+ transients to promote dendrite pruning. We further provide genetic evidence that the local endocytosis in the proximal dendrites functions cooperatively with the global endocytosis-mediated protein degradation mechanism to efficiently promote dendrite pruning. Link between dendritic Ca 2+ transients and thinning We reported that Ca 2+ transients occur in a compartmentalized manner within dendritic branches during early metamorphosis and act as a trigger for dendrite pruning in Drosophila C4da sensory neurons [19] (we hereafter designate the groups of dendrites with compartmentalized Ca 2+ transients as branch units). Since dendritic Ca 2+ transients are typically observed in groups of dendrites distal from the secondary and the tertiary branches ~3 h before the dendrite degeneration [19] , boundary points that compartmentalize the Ca 2+ transients appear to be established at the proximal branches ~3 h before the degeneration of distal dendrites ( Fig. 1g , magenta rectangle region). Previous studies showed that proximal C4da dendrites undergo local changes in membrane structure including thinning and severing of the plasma membrane, as well as cytoskeletal remodelling including destabilization of microtubules and actin filaments, during early metamorphosis [10] , [11] , [12] . We thus investigated the spatial and temporal relationship between these events in the proximal dendrites and the initiation of Ca 2+ transients. To monitor Ca 2+ dynamics and local changes in the plasma membranes or cytoskeletons simultaneously, we expressed both the genetically encoded Ca 2+ indicator GCaMP6s (ref. 20 ) and a red fluorescent reporter (mCD8-RFP to mark plasma membranes, mCherry-α-tubulin to mark microtubules, or lifeact-tdTomato to mark actin filaments) in C4da neurons by taking advantage of the Gal4/UAS system [21] . 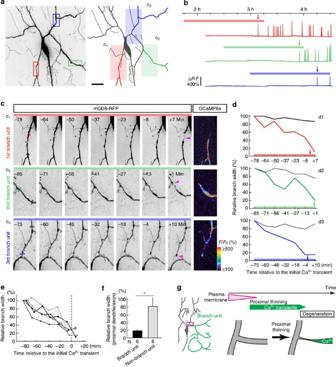Figure 1: Dendrite thinning correlates with Ca2+transients initiation. (a) Live confocal image and corresponding schematic trace of a C4da neuron labelled with mCD8-RFP before the initiation of Ca2+transients (0.5 h a.p.f.). Dendritic branches corresponding future branch units are shown with colours. Three coloured rectangles in the left are the regions from which fluorescent traces of GCaMP6s inbwere obtained. The coloured areas in the right trace (c1 to c3) correspond to the regions shown inc. Scale bar, 20 μm. (b) Time traces of GCaMP6s fluorescence in three different regions, the locations of which are indicated ina. Coloured arrows indicate the first Ca2+transients in each branch unit. The coloured horizontal lines define the time window forc. (c) Time-lapse series of live confocal images of mCD8-RFP fluorescence. Magenta arrowheads indicate the proximal edges of branch units. Time stamps are minutes after the initiation of Ca2+transients. The branch units are visualized with ratiometric images of GCaMP6s. Rectangles correspond to the regions for analyses ind. (d) Time traces of relative branch width in two regions. The corresponding regions are indicated incwith the same colours. (e) Time traces of relative branch width at the boundary of branch units and non-branch units. All the traces are time-aligned to the onset of Ca2+transients. Six regions from four animals are analysed. (f) Quantification of branch width at the proximal dendrites of branch units and non-branch units. *P<0.05; Student’st-test. Error bars, s.e. (g) Schematic diagram showing the temporal and spatial relationship between the proximal thinning and Ca2+transients initiation. Figure 1: Dendrite thinning correlates with Ca 2+ transients initiation. ( a ) Live confocal image and corresponding schematic trace of a C4da neuron labelled with mCD8-RFP before the initiation of Ca 2+ transients (0.5 h a.p.f.). Dendritic branches corresponding future branch units are shown with colours. Three coloured rectangles in the left are the regions from which fluorescent traces of GCaMP6s in b were obtained. The coloured areas in the right trace (c1 to c3) correspond to the regions shown in c . Scale bar, 20 μm. ( b ) Time traces of GCaMP6s fluorescence in three different regions, the locations of which are indicated in a . Coloured arrows indicate the first Ca 2+ transients in each branch unit. The coloured horizontal lines define the time window for c . ( c ) Time-lapse series of live confocal images of mCD8-RFP fluorescence. Magenta arrowheads indicate the proximal edges of branch units. Time stamps are minutes after the initiation of Ca 2+ transients. The branch units are visualized with ratiometric images of GCaMP6s. Rectangles correspond to the regions for analyses in d . ( d ) Time traces of relative branch width in two regions. The corresponding regions are indicated in c with the same colours. ( e ) Time traces of relative branch width at the boundary of branch units and non-branch units. All the traces are time-aligned to the onset of Ca 2+ transients. Six regions from four animals are analysed. ( f ) Quantification of branch width at the proximal dendrites of branch units and non-branch units. * P <0.05; Student’s t -test. Error bars, s.e. ( g ) Schematic diagram showing the temporal and spatial relationship between the proximal thinning and Ca 2+ transients initiation. Full size image An example of long-term simultaneous monitoring of structural changes in the plasma membrane and the occurrence of compartmentalized Ca 2+ transients in single neurons is shown in Fig. 1 . The first branch unit started its Ca 2+ transients at 3 h a.p.f. ( Fig. 1a,b , red arrow). In this branch unit, dendrite thinning at the proximal region became visible ~60 min before the branch unit started Ca 2+ transients, and the relative branch width of the thinning region was reduced to 22.5% of the initial size at the timing when its distal region started Ca 2+ transients ( Fig. 1c,d , red region). Similarly, in the second and the third branch units, proximal dendrite started thinning ~60 min before the Ca 2+ transients in the distal branches and became thinner to ~20% of the initial size, while no obvious thinning was observed in the neighbouring regions ( Fig. 1c,d , compare green and blue regions with black regions). In all neurons we observed, branch units commenced Ca 2+ transients at the timing when their proximal regions become as thin as ~20% of the initial size ( Fig. 1e ; 23.1±9.1%, mean±s.d., n =6 branch units from four animals; compared with 75~84 min before the initiation of Ca 2+ transients). Importantly, no obvious Ca 2+ transients were detected in dendritic branches that did not have significant thinning in the proximal regions ( Fig. 1f ). These data indicate a strong correlation in location and timing between dendrite thinning and Ca 2+ transients and suggest a possible role of dendrite thinning in induction of Ca 2+ transients in branch units ( Fig. 1g ). In contrast to the tight spatiotemporal correlation between dendrite thinning and Ca 2+ transients, microtubule disruption was observed throughout the proximal regions of the dendrite arbor: over 50% of the local disruption in microtubules was observed in dendritic regions that had not experienced any Ca 2+ transients yet ( Supplementary Fig. 1 ; 57% of microtubule-disrupted regions, n =42 regions from six animals), implying that microtubule disruption might act as a permissive rather than an inductive factor for Ca 2+ transients. Indeed, in most cases (14/16 observed neurons), microtubules were disrupted in the proximal regions of branch units before the initiation of Ca 2+ transients with a varying time lag (76.4±39.3 min, mean±s.d.). In addition, actin filaments were still visible around the boundaries including thinning regions ( Supplementary Fig. 1 , 92%, n =26 branch units from 10 animals). Dendrite thinning compartmentalizes pruning dendrites To investigate the role of dendrite thinning in compartmentalization of pruning dendrites, we performed photoactivation experiments using a photoactivatable red fluorescent protein TagRFP (PA-TagRFP [22] ) in parallel with Ca 2+ imaging ( Fig. 2a ). We photoactivated PA-TagRFP in the soma of C4da neurons that just commenced the compartmentalized Ca 2+ transients and found that fluorescent PA-TagRFP proteins were no longer diffused over the thinning region between branch units and non-branch units ( Fig. 2b,c , green open arrowheads). In contrast, fluorescent PA-TagRFP proteins diffused into the dendritic branches without Ca 2+ transients, although the diffusion became slower in some dendrites that were likely in the process of proximal thinning ( Fig. 2c,d , region 2, and Supplementary Movie 1 ). Throughout our experiments, we never observed any diffusion of PA-TagRFP into branch units ( n =15 branch units), while PA-TagRFP proteins diffused into most dendritic branches without Ca 2+ transients (88% of cases, n =42 non-branch units; 16 animals in total were examined). In addition, fluorescence recovery after photobleaching (FRAP) experiments demonstrated that protein diffusion (green fluorescent protein (GFP) in this case) was also inhibited from the branch unit into non-branch units ( Supplementary Fig. 2 ). These data indicate that dendrite thinning provides bidirectional diffusion barriers for cytosolic components at the boundaries between branch units and non-branch units, and raise a possibility that dendrite thinning might contribute to compartmentalization of dendritic Ca 2+ transients ( Fig. 1g ). 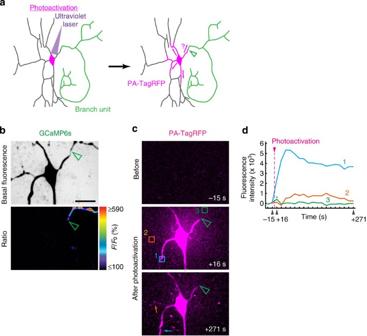Figure 2: Proximal thinning prevents protein diffusion. (a) A schematic of the photoactivation experiment. The cell body of C4da neurons expressing PA-TagRFP is photoactivated with ultraviolet laser, just after they commence compartmentalized Ca2+transients. Distal diffusion of photoactivated PA-TagRFP is monitored after the photoactivation. (b) Representative images of a C4da neuron expressing GCaMP6s. Top, basal fluorescence of GCaMP6s in a C4da neuron. Bottom, a ratiometric image of GCaMP6s fluorescence showing the robust Ca2+influx into a branch unit. Both images are taken just before photoactivation. Green open arrowheads indicate the proximal edge of the branch unit. Scale bar, 20 μm. (c) Representative images showing distal diffusion of photoactivated PA-TagRFP. Time stamps are seconds after the photoactivation. The regions for quantitative analysis indare shown in the middle panel. Arrows indicate the diffusion of PA-TagRFP into non-branch unit. Sixteen animals in total were examined. (d) Time course of PA-TagRFP diffusion in the dendritic regions. Regions of interest are shown inc. An asterisk indicates artificial increase of the red fluorescence around the cell body after photoactivation. Figure 2: Proximal thinning prevents protein diffusion. ( a ) A schematic of the photoactivation experiment. The cell body of C4da neurons expressing PA-TagRFP is photoactivated with ultraviolet laser, just after they commence compartmentalized Ca 2+ transients. Distal diffusion of photoactivated PA-TagRFP is monitored after the photoactivation. ( b ) Representative images of a C4da neuron expressing GCaMP6s. Top, basal fluorescence of GCaMP6s in a C4da neuron. Bottom, a ratiometric image of GCaMP6s fluorescence showing the robust Ca 2+ influx into a branch unit. Both images are taken just before photoactivation. Green open arrowheads indicate the proximal edge of the branch unit. Scale bar, 20 μm. ( c ) Representative images showing distal diffusion of photoactivated PA-TagRFP. Time stamps are seconds after the photoactivation. The regions for quantitative analysis in d are shown in the middle panel. Arrows indicate the diffusion of PA-TagRFP into non-branch unit. Sixteen animals in total were examined. ( d ) Time course of PA-TagRFP diffusion in the dendritic regions. Regions of interest are shown in c . An asterisk indicates artificial increase of the red fluorescence around the cell body after photoactivation. Full size image To further test this possibility, we next explored the relationship between dendrite thinning and elevation of branch excitability, the first sign of compartmentalization of pruning dendrites, which is detected before the initiation of Ca 2+ transients and presumably facilitates compartmentalized Ca 2+ transients via the voltage-gated calcium channels (VGCCs) [19] . As reported previously, we expressed channelrhodopsin-2 (ref. 23 ) fused with GFP (ChR2-EGFP) and red fluorescent calcium indicator RGECO1 (ref. 24 ) in C4da neurons, and stimulated them with blue light pulses to induce VGCCs-mediated Ca 2+ influx into dendrites ( Fig. 3a ). By changing the intensity of blue light, we determined the threshold intensity for the light-induced Ca 2+ influx, which reflects intrinsic excitability of the dendritic branches [19] . We repeated photostimulation experiments against the same neurons and found that local elevation of branch excitability was typically detected at the time when marked proximal thinning was observed selectively at the boundary between dendrites with the unchanged and the elevated intrinsic excitability ( Fig. 3b–d , see green region; 25.9±4.4% of the original branch width, mean±s.e.m., n =4 regions from four animals). In all cases we observed, proximal regions of dendrites with elevated excitability became significantly thinner compared with other regions in the same neurons ( Fig. 3e , relative branch width of proximal regions: dendrites with increased excitability, 18.7±1.7%; dendrite with normal excitability, 84.7±12.6%; mean±s.e.m., n =5 regions for each). Therefore, our data suggest that branch thinning in the proximal dendrites induces local elevation of branch excitability in their distal regions, which thus presumably promotes the robust VGCCs-mediated Ca 2+ influx in branch units. 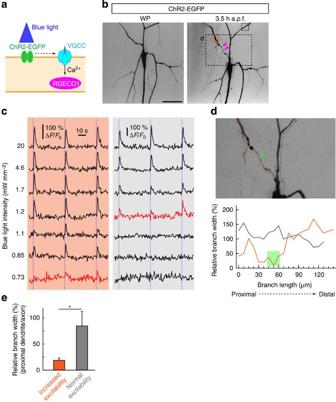Figure 3: Proximal thinning defines dendrites with higher excitability. (a) A schematic of the photostimulation experiment. In C4da neurons expressing channelrhodopsin-2 fused with GFP (ChR2-EGFP), blue light pulses drive concomitant VGCCs-mediated Ca2+responses in dendrites, which are detected by the Ca2+indicator RGECO1, depending on the stimulation light intensity. (b) Live confocal images of an identical neuron at the white pupal stage (left, WP) and 3.5 h a.p.f. (right) labelled with channelrhodopsin-2 fused with GFP (ChR2-EGFP). Magenta arrowheads mark the proximal dendrites with thinning. Orange and grey squares correspond to the regions from which fluorescent traces of RGECO1 incwere obtained. Scale bar, 100 μm. (c) RGECO1 fluorescence changes in response to various intensities of blue light. Time traces obtained from the orange and grey square regions inbat 3.5 h a.p.f. are shown on the left and right, respectively. Traces at the threshold intensities of blue light for inducing dendritic Ca2+responses are indicated in red. The threshold intensity was lower in the orange region (0.73 mW mm−2) compared with that in the grey region (1.2 mW mm−2), indicating that intrinsic excitability is elevated by a factor of 2 in the orange region (that is, dendrites distal from the thinning region). Note that no ‘spontaneous’ Ca2+transients were generated during the photostimulation experiments, indicating that compartmentalized Ca2+transients had not started yet. (d) Quantification of dendritic branch width at the proximal edge of dendrites with elevated excitability. Top, a live confocal image corresponding to a dashed rectangle inb. The proximal edge of dendrites with elevated excitability is shown with a green line. Quantification was done along dashed arrows. Values are relative to an unthinned dendritic region in the same neuron. Representative result from five experiments is shown ina–d. (e) Quantification of branch width at the proximal regions of dendrites with (orange) and without (grey) increased excitability. Ten single dendrites were analysed. *P<0.01;t-test. Error bars, s.d. Figure 3: Proximal thinning defines dendrites with higher excitability. ( a ) A schematic of the photostimulation experiment. In C4da neurons expressing channelrhodopsin-2 fused with GFP (ChR2-EGFP), blue light pulses drive concomitant VGCCs-mediated Ca 2+ responses in dendrites, which are detected by the Ca 2+ indicator RGECO1, depending on the stimulation light intensity. ( b ) Live confocal images of an identical neuron at the white pupal stage (left, WP) and 3.5 h a.p.f. (right) labelled with channelrhodopsin-2 fused with GFP (ChR2-EGFP). Magenta arrowheads mark the proximal dendrites with thinning. Orange and grey squares correspond to the regions from which fluorescent traces of RGECO1 in c were obtained. Scale bar, 100 μm. ( c ) RGECO1 fluorescence changes in response to various intensities of blue light. Time traces obtained from the orange and grey square regions in b at 3.5 h a.p.f. are shown on the left and right, respectively. Traces at the threshold intensities of blue light for inducing dendritic Ca 2+ responses are indicated in red. The threshold intensity was lower in the orange region (0.73 mW mm −2 ) compared with that in the grey region (1.2 mW mm −2 ), indicating that intrinsic excitability is elevated by a factor of 2 in the orange region (that is, dendrites distal from the thinning region). Note that no ‘spontaneous’ Ca 2+ transients were generated during the photostimulation experiments, indicating that compartmentalized Ca 2+ transients had not started yet. ( d ) Quantification of dendritic branch width at the proximal edge of dendrites with elevated excitability. Top, a live confocal image corresponding to a dashed rectangle in b . The proximal edge of dendrites with elevated excitability is shown with a green line. Quantification was done along dashed arrows. Values are relative to an unthinned dendritic region in the same neuron. Representative result from five experiments is shown in a – d . ( e ) Quantification of branch width at the proximal regions of dendrites with (orange) and without (grey) increased excitability. Ten single dendrites were analysed. * P <0.01; t -test. Error bars, s.d. Full size image Endocytic activity is locally elevated in proximal dendrites Given that local and dynamic plasma membrane deformations in neuronal branches are often associated with membrane trafficking events such as endocytosis [25] , [26] , [27] , we reasoned that endocytosis might be recruited in the proximal dendrites to allow for local changes in the plasma membrane structure. To monitor endocytic activity in single dendrites, we utilized a genetically encoded reporter using a pH-sensitive green fluorescent protein (ecliptic pHluorin), in which an ecliptic pHluorin is inserted in the extracellular amino-terminal region of a red fluorescent plasma membrane marker CD4-tdTomato [28] ( Fig. 4a ). Since ecliptic pHluorin is protonated and its fluorescence is largely quenched in the low-pH environment such as inside endocytic compartments [29] , pHluorin-CD4-tdTomato is both green and red fluorescent when localized in the cell surface, whereas green fluorescence is lost when the marker is internalized into acidic endosomes. 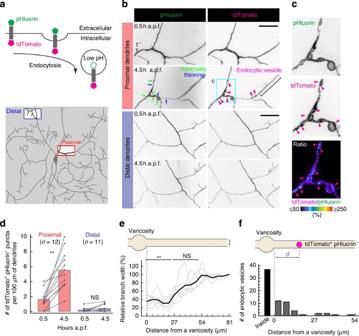Figure 4: Local elevation of endocytic activity in proximal dendrites. (a) Top, schematic diagram of the membrane topology of pHluorin-CD4-tdTomato in the endocytic pathway. Fluorescent and non-fluorescent pHluorin are indicated with filled and open pentagons, respectively. Bottom, dendritic regions observed by high-magnification imaging. (b) Representative images of the proximal and distal dendrites of C4da neurons expressing pHluorin-CD4-tdTomato (from 12 and 11 experiments, respectively). For each region, images are taken from the same branches at 0.5 and 4.5 h a.p.f. Green arrows, varicosities; blue arrows, thin regions; magenta arrowheads, tdTomato+pHluorin−endocytic vesicles; an open arrowhead, the primary dendrite; and a bracket, a dendritic region with no apparent structural changes during the imaging period. Scale bars, 20 μm. (c) High-magnification images of a boxed area inb. A ratiometric image by dividing the image of the green channel by that of the red channel is shown in the bottom. (d) Quantification of the number of tdTomato+pHluorin−endocytic vesicles in the proximal and distal dendrites at 0.5 and 4.5 h a.p.f. **P<0.001, pairedt-test. NS, not significant. (e) Quantification of dendritic branch width in relation to the distance from varicosities. The thick line corresponds to the average of individual branches (grey). **P<0.05, Tukey’s test: compared with branch width at 54 μm from a varicosity (n=6 dendrites). (f) Histogram of the number of endocytic vesicles in relation to the distance from varicosities (n=71 vesicles). Figure 4: Local elevation of endocytic activity in proximal dendrites. ( a ) Top, schematic diagram of the membrane topology of pHluorin-CD4-tdTomato in the endocytic pathway. Fluorescent and non-fluorescent pHluorin are indicated with filled and open pentagons, respectively. Bottom, dendritic regions observed by high-magnification imaging. ( b ) Representative images of the proximal and distal dendrites of C4da neurons expressing pHluorin-CD4-tdTomato (from 12 and 11 experiments, respectively). For each region, images are taken from the same branches at 0.5 and 4.5 h a.p.f. Green arrows, varicosities; blue arrows, thin regions; magenta arrowheads, tdTomato + pHluorin − endocytic vesicles; an open arrowhead, the primary dendrite; and a bracket, a dendritic region with no apparent structural changes during the imaging period. Scale bars, 20 μm. ( c ) High-magnification images of a boxed area in b . A ratiometric image by dividing the image of the green channel by that of the red channel is shown in the bottom. ( d ) Quantification of the number of tdTomato + pHluorin − endocytic vesicles in the proximal and distal dendrites at 0.5 and 4.5 h a.p.f. ** P <0.001, paired t -test. NS, not significant. ( e ) Quantification of dendritic branch width in relation to the distance from varicosities. The thick line corresponds to the average of individual branches (grey). ** P <0.05, Tukey’s test: compared with branch width at 54 μm from a varicosity ( n =6 dendrites). ( f ) Histogram of the number of endocytic vesicles in relation to the distance from varicosities ( n =71 vesicles). Full size image To examine the spatial relationship between endocytic activity and dendritic branch thinning, we expressed pHluorin-CD4-tdTomato in C4da neurons and observed the proximal and distal dendrites separately at high magnification from the onset of metamorphosis ( Fig. 4a,b ). We noted little difference in fluorescence patterns between pHluorin and tdTomato along distal dendrites, where no obvious dendrite thinning was detectable throughout the imaging period ( Fig. 4b,d ). Similarly, little difference between the tdTomato and pHluorin fluorescence was noted in the proximal dendrites at 0.5 h a.p.f. ( Fig. 4b,d ). Within the next 4 h, however, we noted significant localized differences in tdTomato and pHluorin fluorescence: some proximal branches showed varicosities ( Fig. 4b , green arrows), around which dendrites were extremely thin compared with other regions ( Fig. 4b , blue arrows) and intracellular dotted structures with tdTomato signal but without pHluorin signal (tdTomato + pHluorin − ) were evident in these regions ( Fig. 4b,c , magenta arrowheads), suggestive of increased local endocytic activity. Most of these dotted structures in the proximal dendrites were likely to be the endocytic compartments including early endosomes, based on the following observations: first, when we expressed the plasma membrane marker CD4-tdTomato in C4da neurons, similar dotted structures were detected specifically in the thinning dendrites, but not in the unthinned regions ( Supplementary Fig. 3 ). Second, 75% of the dotted structures were co-localized with the early endosome marker 2xFYVE-GFP [30] ( Supplementary Fig. 3 , n =129 dots from four animals). To our interest, such dotted structures were present mostly at the boundaries of the thinned regions of proximal dendrites ( Fig. 4b , bracket: proximal dendrites just distal from the boundary that show no tdTomato + pHluorin − dots), suggesting a close spatial relationship between the elevated endocytic activity and dendrite thinning. To further confirm this, we quantified the spatial relationship between dendrite thinning, varicosity formation and endocytic activity ( Fig. 4e,f ). These analyses revealed a tight spatial relationship between dendrite thinning and varicosity formation, as dendritic branches were significantly thinner around varicosities ( Fig. 4e ) as well as between the endocytic vesicles and the thinning regions, as the closer to varicosities, the more dendritic tdTomato + pHluorin − dots were detected ( Fig. 4f ). Taken together, these observations demonstrate a spatial correlation between local endocytic activity, varicosity formation and dendrite thinning. To more precisely investigate the temporal relationship between endocytic activity and branch thinning in the proximal dendrites, we performed time-lapse imaging experiments to continuously and simultaneously follow early endosome formation and plasma membrane deformation from the onset of metamorphosis by visualizing 2xFYVE-GFP and mCD8-RFP, respectively. The FYVE domain binds to phosphatidylinositol 3-phosphate, which is generated on endosomal membranes by a phosphatidylinositol 3-kinase [31] . The fluorescent intensity of 2xFYVE-GFP puncta, which therefore reflects phosphatidylinositol 3-phosphate levels on early endosomes, increases progressively when newly endocytosed vesicles progress along the endocytic pathway to form early endosomes [32] . Hence, we hypothesized that if local endocytosis induces the proximal thinning, progressive increase in the green fluorescence should be observed in a time-correlated manner with it. An example of long-term simultaneous monitoring of 2xFYVE-GFP puncta and plasma membrane structures is shown in Fig. 5 . From 1.5 to 3 h a.p.f., we observed dim 2xFYVE-GFP puncta, some of which were mobile and travelled in a distal-to-proximal direction, as evident by weak diagonal lines in the kymograph ( Fig. 5a,b , open arrowheads between t 0 and t 1 ). During this observation period, little structural changes were noted in the proximal dendrites ( Fig. 5c,d ). At 3 h a.p.f., in contrast, bright and relatively stationary fluorescent signals started to appear in the proximal regions ( Fig. 5c , magenta arrowheads after t 2 ). This is evident by strong horizontal lines in the kymograph ( Fig. 5b , see white arrowheads). We noted that the plasma membrane structure changed progressively in these regions from~3 h a.p.f. : dendritic branches became thinner and varicosities appeared around the thinning regions ( Fig. 5c,d , blue and green arrows). In contrast, no such structural changes were observed in the plasma membrane of the regions where little increase in 2xFYVE-GFP was observed ( Fig. 5c,d ). Similar results were obtained in all nine C4da neurons analysed, suggesting that structural changes in the plasma membrane occurred in a time-correlated manner with the appearance of bright 2xFYVE-GFP puncta. Interestingly, fine tracking of single vesicles revealed that many 2xFYVE-GFP puncta formed in the proximal dendrites were quickly incorporated into varicosities, which increased in volume as nearby branches became progressively thinner ( Fig. 5e , see time-lapse series of images taken at 4 h a.p.f., and Supplementary Movie 2 ). These observations further support the model in which local endocytosis contributes to dendrite thinning as well as varicosity formation in the proximal dendrites ( Fig. 5f ). 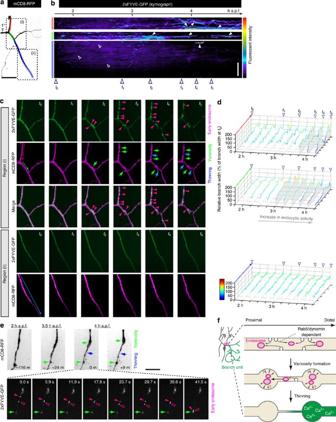Figure 5: Endosome formation correlates with proximal thinning. (a) A confocal image of the proximal dendrites visualized with mCD8-RFP. Dendritic branches traced in red, green and blue correspond to those analysed inb. Regions (i) and (ii) correspond to those analysed inc. An open arrowhead indicates the primary dendrite. Scale bar, 20 μm. (b) Representative 2xFYVE-GFP kymographs in three dendritic branches traced ina. Open arrowheads, dim and mobile puncta; and white arrowheads, bright and stationary puncta. Scale bar, 20 μm. (c) Live confocal images of 2xFYVE-GFP and mCD8-RFP at six different time points (indicated with blue open arrowheads inb). Magenta arrowheads, 2xFYVE-GFP positive early endosomes; green arrows, varicosities; and blue arrows, thin regions. Dashed arrows indicate the dendritic regions analysed ind. (d) Time course of branch thinning in relation to the increase in endocytic activity. The values are relative to the branch width at time t0. Relative branch width is represented by thezaxis and with colours. Areas beneath the traces are filled with grey colour, after bright and stationary 2xFYVE-GFP puncta have emerged (that is, endocytic activity has increased). A representative neuron from nine independent experiments is shown ina–d. (e) Time-lapse series of live confocal images of mCD8-RFP and 2xFYVE-GFP fluorescence. Two 2xFYVE-GFP positive early endosomes (filled and open magenta arrowheads) are incorporated into a varicosity (a green arrow). See alsoSupplementary Movie 2for the entire set of time-lapse images. Blue arrows, thinning dendritic branches. Scale bar, 10 μm. Another representative neuron is analysed ine. (f) Proposed model of local endocytosis-mediated compartmentalization of Ca2+signaling in C4da dendrite pruning. Endocytosis occurs locally in the proximal dendrites to form endocytic vesicles, which are actively transported into the nearby varicosities. Membrane components might be redelivered to the plasma membrane in the varicosities to increase their volume. This could result in decrease of membranes in the thinning dendrites (see also Discussion). Figure 5: Endosome formation correlates with proximal thinning. ( a ) A confocal image of the proximal dendrites visualized with mCD8-RFP. Dendritic branches traced in red, green and blue correspond to those analysed in b . Regions (i) and (ii) correspond to those analysed in c . An open arrowhead indicates the primary dendrite. Scale bar, 20 μm. ( b ) Representative 2xFYVE-GFP kymographs in three dendritic branches traced in a . Open arrowheads, dim and mobile puncta; and white arrowheads, bright and stationary puncta. Scale bar, 20 μm. ( c ) Live confocal images of 2xFYVE-GFP and mCD8-RFP at six different time points (indicated with blue open arrowheads in b ). Magenta arrowheads, 2xFYVE-GFP positive early endosomes; green arrows, varicosities; and blue arrows, thin regions. Dashed arrows indicate the dendritic regions analysed in d . ( d ) Time course of branch thinning in relation to the increase in endocytic activity. The values are relative to the branch width at time t 0 . Relative branch width is represented by the z axis and with colours. Areas beneath the traces are filled with grey colour, after bright and stationary 2xFYVE-GFP puncta have emerged (that is, endocytic activity has increased). A representative neuron from nine independent experiments is shown in a – d . ( e ) Time-lapse series of live confocal images of mCD8-RFP and 2xFYVE-GFP fluorescence. Two 2xFYVE-GFP positive early endosomes (filled and open magenta arrowheads) are incorporated into a varicosity (a green arrow). See also Supplementary Movie 2 for the entire set of time-lapse images. Blue arrows, thinning dendritic branches. Scale bar, 10 μm. Another representative neuron is analysed in e . ( f ) Proposed model of local endocytosis-mediated compartmentalization of Ca 2+ signaling in C4da dendrite pruning. Endocytosis occurs locally in the proximal dendrites to form endocytic vesicles, which are actively transported into the nearby varicosities. Membrane components might be redelivered to the plasma membrane in the varicosities to increase their volume. This could result in decrease of membranes in the thinning dendrites (see also Discussion). Full size image Local endocytosis involves Rab5 and dynamin Previous studies suggest that distinct endocytosis pathways coexist in a cell, which are largely classified through their differential dependencies on certain regulators including Rab5, dynamin, Arf6 and Flotillin [33] . To gain molecular insights into the endocytic pathways that are involved in this localized dendrite thinning, we inhibited each endocytic pathway by expressing dominant negative forms or short hairpin RNAs (shRNAs) for these regulators in C4da neurons, and monitored the endocytic activity by pHluorin-CD4-tdTomato. In C4da neurons expressing the dominant negative Arf6 (Arf6-DN) or shRNA for Flotillin, we found that both formation of the tdTomato + pHluorin − puncta and dendritic thinning occurred normally in the proximal regions at 4 h a.p.f. ( Supplementary Fig. 4 ). In contrast, expression of a dominant negative form of Rab5 (Rab5-DN) resulted in marked defects in both events ( Supplementary Fig. 4 ). Similar defects were obtained by the overexpression of a dominant negative form of Shibire (Shi), the fly homologue of dynamin ( Supplementary Fig. 4 ). Importantly, blocking neither Rab5 nor Shi function in C4da neurons prevented the microtubule destabilization in proximal dendrites ( Supplementary Fig. 5 ). These data suggest that blocking this endocytic pathway did not broadly inhibit all the cellular events associated with pruning but instead had a targeted effect on localized membrane thinning that precedes formation of Ca 2+ transients and dendrite severing. Taken together, these data suggest that Rab5- and dynamin-dependent local endocytosis in the proximal dendrites is required for dendrite thinning but not for microtubule destabilization. Given that Rab5- and dynamin-dependent endocytosis is required for the dendrite thinning, we next asked whether Rab5- and dynamin-dependent endocytosis might contribute to the compartmentalized Ca 2+ transients in dendritic branches. We found that the expression of Rab5-DN or Shi-DN significantly reduced the number of C4da neurons exhibiting Ca 2+ transients at 7 h a.p.f., when compartmentalized Ca 2+ transients were typically observed in control neurons ( Fig. 6a,b ). By contrast, blocking Arf6 or Flotillin activity had little effect on appearance of Ca 2+ transients ( Fig. 6b ). These data suggest that Rab5- and dynamin-dependent local endocytosis is required for defining C4da dendrites into branch units. 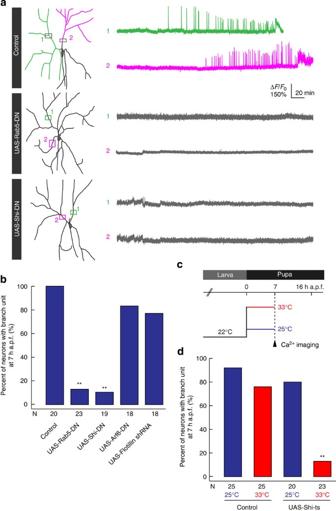Figure 6: Rab5 and dynamin are required for Ca2+transients initiation. (a) Long-term time traces of GCaMP6s fluorescence in control (top), Rab5-DN expressing (middle) and Shi-DN expressing neurons (bottom). Fluorescence changes in two rectangle regions are shown. (b) Quantification of the percentage of C4da neurons with dendrites producing Ca2+transients at 7 h a.p.f.. **P<0.001,χ2-test followed by Ryan’s test. (c) Scheme of the temperature shift experiment. Animals expressing or not expressing Shi-ts in C4da neurons are raised at 22 °C during the entire larval stage, and at the permissive (25 °C) or non-permissive (33 °C) temperature from the onset of metamorphosis. Ca2+imaging is performed at 7 h a.p.f.. (d) Quantification of the percentage of C4da neurons with dendrites producing Ca2+transients at 7 h a.p.f.. **P<0.001 comparing with all other groups, Fisher’s exact test. Figure 6: Rab5 and dynamin are required for Ca 2+ transients initiation. ( a ) Long-term time traces of GCaMP6s fluorescence in control (top), Rab5-DN expressing (middle) and Shi-DN expressing neurons (bottom). Fluorescence changes in two rectangle regions are shown. ( b ) Quantification of the percentage of C4da neurons with dendrites producing Ca 2+ transients at 7 h a.p.f.. ** P <0.001, χ 2 -test followed by Ryan’s test. ( c ) Scheme of the temperature shift experiment. Animals expressing or not expressing Shi-ts in C4da neurons are raised at 22 °C during the entire larval stage, and at the permissive (25 °C) or non-permissive (33 °C) temperature from the onset of metamorphosis. Ca 2+ imaging is performed at 7 h a.p.f.. ( d ) Quantification of the percentage of C4da neurons with dendrites producing Ca 2+ transients at 7 h a.p.f.. ** P <0.001 comparing with all other groups, Fisher’s exact test. Full size image In the above experiments, it is unclear whether endocytosis is required at the time of dendrite pruning, because the dominant negative proteins were expressed in C4da neurons from the beginning of larval development. It is thus possible that the defects in the occurrence of dendritic Ca 2+ transients could be secondary to interference with endocytosis before dendrite pruning (that is, during larval stages [34] ). To perturb dynamin-dependent endocytosis in C4da neurons only from the onset of the pupal stage, we utilized the targeted expression of a temperature-sensitive shibire (Shi-ts), which acutely prevents dynamin-dependent endocytosis at the non-permissive temperature (33 °C) [35] ( Fig. 6c ). In control animals, Ca 2+ transients occurred normally both at the permissive (25 °C) and non-permissive (33 °C) temperature ( Fig. 6d ). No obvious defects in the occurrence of Ca 2+ transients were observed in pupae expressing Shi-ts that were raised at the permissive temperature throughout development ( Fig. 6d ). However, when animals expressing Shi-ts in C4da neurons were raised at the permissive temperature during the entire larval stage and were shifted to the non-permissive temperature from 0 h a.p.f., the number of C4da neurons exhibiting Ca 2+ transients was significantly reduced at 7 h a.p.f. ( Fig. 6d ). Thus, dynamin-dependent endocytosis is required in the pupal stage to drive compartmentalized Ca 2+ transients. Two distinct endocytic mechanisms promote dendrite pruning It was recently reported that Rab5-dependent endocytosis promotes dendrite pruning through degradation of the cell surface molecule Neuroglian (Nrg) and that Nrg uptake from the cell surface is likely to be mediated by global endocytosis in entire neurons since Nrg downregulation was detected in entire neurons including axon, dendrites and the soma [36] . To examine whether the endocytosis-mediated Nrg degradation is required for the dendritic Ca 2+ transients, we investigated the effects of Nrg overexpression on the dendritic Ca 2+ transients during pruning, since Nrg overexpression caused a significant delay of Nrg degradation and thus a significant defect in dendrite pruning [36] . We found that appearance of the dendritic Ca 2+ transients were slightly but not significantly affected by overexpressing Nrg in C4da neurons ( Supplementary Fig 6 ). Consistently, no significant defect in Ca 2+ transients was observed by inhibiting Vps32, the key regulator of Nrg degradation by endocytosis [36] ( Supplementary Fig. 6 ). Thus, global endocytosis-dependent Nrg degradation is dispensable for occurrence of the dendritic Ca 2+ transients. We next examined genetically how the local and the global endocytosis pathways contribute to dendrite pruning by manipulating dendritic Ca 2+ transients and Nrg degradation, which are the downstream outcomes of the local and the global endocytosis pathways, respectively. As shown in Fig. 7 , pruning defects in ca-beta mutant neurons, in which the VGCC activity and thus the dendritic Ca 2+ transients are abolished during pruning [19] , were significantly enhanced by Nrg overexpression, compared with either those in ca-beta mutant neurons or Nrg-overexpressing neurons ( Fig. 7a,b ). Similarly, pruning defects obtained by the overexpression of Kir2.1, which attenuates VGCCs activites [19] , were significantly enhanced by co-expression of a shRNA of Vps32 ( Fig. 7c ). Thus, impairment of both Ca 2+ transients generation (local endocytosis pathway) and Nrg degradation (global endocytosis pathway) resulted in synergistic defects in dendrite pruning. Importantly, the enhanced defects by inhibiting both pathways were comparable to those obtained by the expression of Rab5-DN or Shi-DN (or Shi-ts at non-permissive temperature; Supplementary Fig. 7 ), suggesting these two GTPases regulate both of the local and the global endocytic pathways to promote dendrite pruning. These data support the model that the local endocytosis in the proximal dendrites and the global endocytosis in entire neurons cooperatively promote dendrite pruning, presumably through dendritic Ca 2+ transients and Nrg degradation, respectively ( Fig. 7d ). 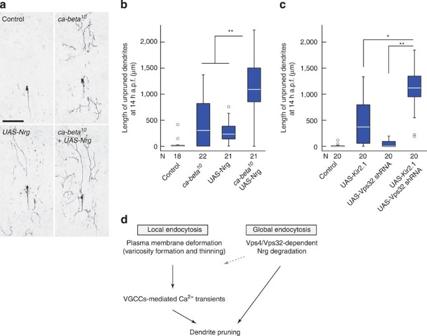Figure 7: Two endocytic pathways cooperatively promote dendrite pruning. (a) Representative images of C4da neurons taken at 14 h a.p.f.. Dendrites are visualized with mCD8-GFP. Scale bar, 100 μm. (b) Quantification of the pruning phenotype in control andca-betamutant neurons overexpressing Nrg. Box plots indicate the median (white line), 25th/75th percentiles (box), the data range except for outliers (whiskers), and outliers (circles). **P<0.001, Steel–Dwass test. (c) Quantification of the pruning phenotype in neurons expressing either Kir2.1 or Vps32 shRNA, or both. *P=0.007, **P<0.001, Steel–Dwass test. (d) The local endocytosis in the proximal dendrite induces deformation of plasma membrane (varicosity formation and dendrite thinning), which is likely to contribute to compartmentalization of VGCCs-mediated Ca2+transients. In parallel, the global endocytosis occurs early in metamorphosis to degrade the cell surface molecule Nrg in a Vps4/Vps32-dependent manner. These two endocytic mechanisms likely promote dendrite pruning in a cooperative manner (see Discussion for details). Since dendritic Ca2+transients were detected precociously innrgmutant neurons36, global endocytosis might possibly have some minor influence on the initiation of Ca2+transients (dashed arrow). Figure 7: Two endocytic pathways cooperatively promote dendrite pruning. ( a ) Representative images of C4da neurons taken at 14 h a.p.f.. Dendrites are visualized with mCD8-GFP. Scale bar, 100 μm. ( b ) Quantification of the pruning phenotype in control and ca-beta mutant neurons overexpressing Nrg. Box plots indicate the median (white line), 25th/75th percentiles (box), the data range except for outliers (whiskers), and outliers (circles). ** P <0.001, Steel–Dwass test. ( c ) Quantification of the pruning phenotype in neurons expressing either Kir2.1 or Vps32 shRNA, or both. * P =0.007, ** P <0.001, Steel–Dwass test. ( d ) The local endocytosis in the proximal dendrite induces deformation of plasma membrane (varicosity formation and dendrite thinning), which is likely to contribute to compartmentalization of VGCCs-mediated Ca 2+ transients. In parallel, the global endocytosis occurs early in metamorphosis to degrade the cell surface molecule Nrg in a Vps4/Vps32-dependent manner. These two endocytic mechanisms likely promote dendrite pruning in a cooperative manner (see Discussion for details). Since dendritic Ca 2+ transients were detected precociously in nrg mutant neurons [36] , global endocytosis might possibly have some minor influence on the initiation of Ca 2+ transients (dashed arrow). Full size image Precise remodelling of neural circuits requires selective pruning of unnecessary dendritic branches, a process that is achieved through the local activation of pruning machineries in dendrites destined to be pruned. We recently reported that compartmentalized Ca 2+ transients in dendritic branches act as temporal and spatial cues to trigger pruning; yet, how these distinct dendritic domains are defined was unknown [19] . In this report, we have found that local elevation of the endocytic activity in dendrites is tightly linked with compartmentalization of dendritic branches that are destined to be pruned in Drosophila C4da neurons. High-resolution imaging of single dendrites and post hoc quantification analysis revealed that endocytic activity was locally and transiently elevated at the proximal dendrites undergoing branch thinning, a cellular event linked with initiation of compartmentalized Ca 2+ transients. We also found that the two GTPases Rab5 and dynamin are required for the local elevation of endocytic activity, thinning of proximal dendrites and generation of compartmentalized Ca 2+ transients. Taken together, these data are consistent with a model in which the local elevation of endocytic activity drives dendrite thinning in the proximal branches and thus defines the dendrites to be or not to be pruned away. How local endocytosis could contribute to dendrite thinning remains to be elucidated. Recent studies suggest that local endocytosis plays a critical role in remodelling of membrane structures [25] , [26] , [37] . For example, remodelling of the apical surface during epithelial morphogenesis in Drosophila embryo is induced by Rab5- and dynamin-dependent endocytosis [37] . In this case, rapid internalization of the apical plasma membrane likely triggers changes of apical morphology. It appears thus possible that a massive increase in the internalization of the local dendritic membrane could act as a major driving force for dendrite thinning. In addition to the local increase in the endocytic activity, we found that the internalized vesicles in the proximal dendrites often moved into varicosities, which kept increasing in volume, while nearby branches became progressively thinner suggesting that internalized membrane lipids are redelivered to the nearby plasma membrane to facilitate the varicosity formation ( Fig. 5f ). This redelivery might contribute to progressive dendrite thinning without stuck in membrane trafficking. Thus, local endocytosis might contribute not only to dendrite thinning but also to varicosity formation in the proximal dendrites. Consistent with this idea, blockage of dendritic endocytosis caused complete inhibition of varicosity formation. We propose that dendrite thinning promotes pruning, at least in part, through induction of the compartmentalized Ca 2+ transients in branch units. This idea is supported by the following lines of evidence. First, dendrite thinning is spatially and temporally correlated with the initiation of dendritic Ca 2+ transients. Second, photoactivation and FRAP experiments revealed that dendrite thinning likely functions to restrict molecular diffusion into and out of dendritic branches where Ca 2+ transients are induced. Finally, inhibition of the local increase of endocytosis, which resulted in prominent defects in dendrite thinning, impaired the initiation of compartmentalized Ca 2+ transients, but not other events in the proximal dendrites such as destabilization of microtubules. How could dendrite thinning induce Ca 2+ transients in branch units? Our quantification data showed that dendritic branches have a critical threshold in the branch width to commence the dendritic Ca 2+ transients in branch units. This threshold is comparable to the branch width at the boundaries between branches with the unchanged and the elevated branch excitability. It is thus likely that dendrite thinning induces the dendritic Ca 2+ transients by elevating the branch excitability in the distal dendrites. Given that proximal thinning contributes to the formation of molecular diffusion barriers, dendrite thinning might limit supply of cytosolic factors or organelles from the soma to branch units, which might contribute to elevation of the branch excitability. For example, mitochondria are continuously transported from the soma to dendritic branches, which likely supply most part of ATP in dendrites [38] . In most excitable cells, the resting membrane potential is maintained predominantly by Na + /K + ATPases on the plasma membrane, whose activity is highly dependent on the cytosolic ATP levels [39] . It is thus possible that dendrite thinning blocks dendritic transport of mitochondria, regulators of ATP synthesis and/or ATP itself into branch units, which leads to the impairment of Na + /K + ATPases function in branch units, thereby resulting in the local elevation of membrane excitability in branch units. In addition to the induction of Ca 2+ transients, thinning might also contribute to the compartmentalization of Ca 2+ transients by limiting the propagation of voltage signal within dendritic branches. Since the membrane resistance and axial resistance, which depend inversely on the circumference (2 π r , where r is the radius of dendrites) and cross-sectional area (2 π r 2 ) of dendritic branches, respectively, are expected to be much higher in the thinning regions than in the thicker distal regions [40] , the voltage signal travelling along dendritic branches is likely to be attenuated at the thinning regions. Thus, dendrite thinning could function as a barrier for the propagation of the voltage signal that acts as a driving force of Ca 2+ transients. Consistent with this idea, proximal thinning was spatially correlated with the boundaries between the branch units and non-branch units. It is also possible that varicosities nearby the thinning regions might contribute to buffering Ca 2+ influx. These two possible mechanisms are not required to be mutually exclusive and both might contribute to the compartmentalization of Ca 2+ transients. Taken together, endocytosis-mediated dendrite thinning might contribute to both compartmentalization and initiation of Ca 2+ transients in dendrite pruning. Zhang et al. [36] recently reported that endocytosis was required for degradation of the cell surface molecule Nrg, which occurred in entire neurons including axons, dendrites, and the soma, rather than locally in the proximal dendrites. In the present study, we have demonstrated that the endocytosis-mediated Nrg degradation was not necessary for occurrence of Ca 2+ transients. Furthermore, our genetic data indicated that the endocytosis-mediated Nrg degradation pathway shows a synergistic interaction with the local endocytosis-mediated Ca 2+ transient pathway in dendrite pruning. Importantly, the enhanced pruning defects by suppressing both pathways were comparable to those obtained by Rab5-DN or Shi-DN (or Shi-ts) expression, suggesting these two GTPases regulate both of the local and the global endocytic pathways to promote dendrite pruning. Thus, the local endocytosis in the proximal dendrites and the global endocytosis in entire neurons cooperatively promote dendrite pruning, presumably through dendritic Ca 2+ transients and Nrg degradation, respectively. Since inhibition of endocytosis might potentially affect exocytosis in an indirect manner, it is possible that the pruning defects obtained by inhibiting Rab5 or dynamin could be caused by attenuated exocytic trafficking of some kind of ‘eat-me’ signals. However, we believe this possibility unlikely, firstly because knockdown of genes involved in exocytosis in C4da neurons caused no significant defects in dendrite pruning ( Supplementary Table 1 ), and secondly because in Rab5-DN expressing neurons some amount of dendrites that underwent degeneration were normally phagocytosed by epithelial cells ( Supplementary Fig. 8 ). In the developing mammalian brain, large-scale pruning is observed in many neurons including retinal ganglion cells, hippocampal granule cells and visual cortical neurons [2] , [5] . The cellular mechanism of these pruning has not been elucidated due to difficulties for live imaging, but axon tracing studies have revealed an increase in the thinning and swelling of axonal processes to be pruned [41] , which seems to be similar to those observed in C4da dendrite pruning. Notably, molecular mechanisms involved in dendrite pruning in Drosophila C4da neurons share similarities with axon degeneration in mammalian neurons. For instance, in both cases, degeneration requires Ca 2+ influx through VGCCs into axons or dendrites [19] , [42] . In addition, co-activation of the two proteases calpains and caspases is required for both dendrite degeneration in C4da neurons and axon degeneration in the mouse DRG neurons [19] , [43] . Furthermore, in flies overexpressing the causal gene product of the slow Wallerian degeneration mouse in C4da neurons, dendrite pruning was slightly but significantly retarded [15] , [44] . It is thus of interest to examine that the local activation of the Rab5- and dynamin-dependent endocytosis might be involved in the progress of large-scale axon degeneration in pathological conditions in the mammalian nervous system [45] , [46] . Further studies on the role of local endocytosis in dendrite pruning should also help to elucidate molecular and cellular mechanisms underlying axon/dendrite degeneration in the developing nervous system. Fly stocks Mutants and transgenic lines used in this study are as follows: (1) pickpocket ( ppk )-Gal4 (X), (2) UAS-mCherry-α-tubulin (second, Bloomington#25774), (3) UAS-GCaMP6s (second, Bloomington#42746), (4) UAS-mCD8-RFP (X), (5) UAS-mCD8-GFP (X, from a Bloomington LL4 line), (6) UAS-PA-TagRFP (third, this study), (7) UAS-pHluorin-CD4-tdTomato (third, this study), (8) ppk-CD4-tdTomato (second, Bloomington#35844), (9) UAS-2xFYVE-GFP (second, Bloomington#42712), (10) UAS-Rab5-DN (third, this study), (11) UAS-Shi-DN (third, this study), (12) UAS-Arf6-DN, (13) UAS-Flotillin shRNA (third, Bloomington#36700), (14) UAS-Shi-ts (third, Kitamoto stock), (15) shi 2 (Kyoto#106754), (16) UAS-Nrg, (17) UAS-Vps32 shRNA (Bloomington#38305), (18) ca-beta 10 FRT40A [19] and (19) UAS-Kir2.1-GFP. Stock 1 was from Dr Yuh Nung Jan. Stock 16 was from Dr Fengwei Yu. Stocks 6, 7, 10 and 11 were generated in this study (see below for details), and the rest of the stocks were from the Bloomington and Kyoto stock centres. DNA constructs and transgenic flies UAS-Lifeact-tdTomato . An open reading frame of tdTomato was PCR amplified from a plasmid (ptdTomato-C1 Vector, Takara, Japan) using primers one of which contains a DNA sequence encoding the Lifeact domain, and subcloned into the pJFRC-MUH-20xUAS vector [19] . The plasmid was injected into flies carrying an attP docking site, attP2 (BestGene Inc.). The following primers were used: 5′-AACTCTGAATAGATCTATGGGTGTTGCTGATTTAATTAAAAAGTTCGAAAGTATTAGTAAGGAAGAGGGTGATCCTCCAGTTGCTACTATGGTGAGCAAGGGCGAGGAGG-3′ 5′-TAGAGGTACCCTCGAGTTACTTGTACAGCTCGTCCATGCC-3′ UAS-PA-TagRFP . A complementary DNA (cDNA) of PA-TagRFP was PCR amplified from a plasmid (kindly provided by Dr Verkhusha, Albert Einstein College of Medicine) and subcloned into the pJFRC-MUH-20xUAS vector. The plasmid was injected into flies carrying an attP docking site, attP2 (BestGene Inc.). UAS-pHluorin-CD4-tdTomato . Two DNA sequences encoding pHluorin with amino-terminal signal sequences and CD4-tdTomato were first PCR amplified from plasmids, pCI-SEP_NR2A (Addgene#23997) and pDEST-HemmarR (Addgene#31222), respectively. These two fragments were fused by an overlap extension PCR and then subcloned into the pJFRC-MUH-20xUAS vector. The plasmid was injected into flies carrying an attP docking site, attP2 (BestGene Inc.). The following primers were used: 5′-AACTCTGAATAGATCTATGAATCCCAAGAGCGAAGTCCTCATTGCAGCCGTGCTGTTCATGCTGCTGGCCTGCGTCCAGTGTCAAAGTAAAGGAGAAGAACTTTTCACTG-3′ 5′-GCCGCCACCGCTAGCAGTAGCAACTGGAGGATCACCTTTGTATAGTTCATCCATGCCATGTG-3′ 5′-GCTAGCGGTGGCGGCGGAAGTGGAG-3′ 5′-TAGAGGTACCCTCGAGTTAGAGGGCAACTTCATTTTCATAG-3′ UAS-Rab5-DN . The full-length cDNA of Rab5 was first PCR amplified from a cDNA library prepared from the adult head of yw strain. A single S43N mutation was then induced by standard PCR-based site-directed mutagenesis. The resulting PCR fragment was cloned into the pJFRC-MUH-20xUAS vector. The plasmid was injected into flies carrying an attP docking site, VK00005 (BestGene Inc.). The following primers were used (a mutation site is indicated with lower case letters): 5′-AACTCTGAATAGATCTCAAAATGGCAACCACTCCACGCAG-3′ 5′-GTCCGCTGTGGGCAAGaaCTCACTGGTGCTGCGCT-3′ 5′-AGCGCAGCACCAGTGAGttCTTGCCCACAGCGGAC-3′ 5′-TAGAGGTACCCTCGAGTCACTTGCAGCAGTTGTTCGTC-3′ UAS-Shi-DN . Two different isoforms of the full-length cDNA of shibire , corresponding to shi-RL and shi-RM isoforms in FlyBase ( http://flybase.org/reports/FBgn0003392.html ), were first PCR amplified from a cDNA library prepared from the adult head of yw strain, and cloned into the pJFRC-MUH-CeGFP vector, which is a modified version of the pJFRC-MUH (Addgene#26213). A single K44A mutation was then induced by standard PCR-based site-directed mutagenesis. The resulting PCR fragment was subcloned into the pJFRC-MUH-20xUAS vector. The plasmid was injected into flies carrying an attP docking site, attP2 (BestGene Inc.). Similar defects in dendrite pruning were obtained by expressing dominant negative forms of either isoform (data not shown). All presented data were from experiments using a dominant negative form of shi-RM isoform. The following primers were used (a mutation site is indicated with lower case letters): 5′-AACTCTGAATAGATCTATGGATAGTTTAATTACAATTG-3′ 5′-TAGAGGTACCCTCGAGTTACTTGAATCGCGAACTGAAGGC-3′ 5′-TAGAGGTACCCTCGAGTTAACGACGCGATGGTAGCATTGG-3′ 5′-CAGTCAGCTGGCgcGAGTTCCGTTTTGGAG-3′ 5′-CTCCAAAACGGAACTCgcGCCAGCTGACTG-3′ QUAS-RGECO1 . The codon optimized RGECO1 (ref. 19 ) was PCR amplified and subcloned into the pQUAST plasmid (Addgene#24349). The resulting plasmid was injected into y w strains to obtain transgenics (BestGene Inc.). The following primers were used: 5′-AGGGAATTGGGAATTCCAAAATGGTGGATAGCAGCCGC-3′ 5′-ACAAAGATCCTCTAGATTACTTGGCGGTCATCATCTGC-3′ QUAS-hChR2-EGFP . A variant of channelrhodopsin-2 (H134R) and EGFP were separately PCR amplified, fused by overlap extension PCR, and then subcloned into the pQUAST plasmid. The resulting plasmid was injected into y w strains to obtain transgenics (BestGene Inc.). The following primers were used (the lower case letters correspond to a linker between channelrhodopsin-2 and EGFP): 5′-ATTCGTTAACAGATCTATGGACTATGGCGGCGCTTTGTC-3′ 5′-TAGAGGTACCCTCGAGTTACTTGTACAGCTCGTCCATGC-3′ 5′-GAGGCCGGAGCCGTGCCAggtggaATGGTGAGCAAGGGCGAG-3′ 5′-CTCGCCCTTGCTCACCATtccaccTGGCACGGCTCCGGCCTC-3′ Live imaging experiments Live imaging experiments, except for pruning phenotype analysis, were performed with the following two upright microscopes; Nikon ECLIPSE 90i (Plan Apo objective, × 40 NA=1.0, Nikon), equipped with a spinning-disk confocal unit Yokogawa CSU10 (Yokogawa, Tokyo, Japan) and an electron-multiplying charge-coupled device (EM-CCD) digital camera (iXon, Andor); and Olympus BX51WI (UPlanSApo objective, × 20 NA=0.75; UPLSAPO 60XO objective, × 60 NA=1.35; UPLSAPO 100XO objective × 100 NA=1.4), equipped with a CSU10 spinning-disk confocal system and an EM-CCD digital camera (Evolve, Photometrics). Obtained images were analysed using Metamorph (Molecular Devises) and Image J software ( http://rsb.info.nih.gov/ij/ ) to generate ratiometric images. In the quantification analyses of endocytic vesicles in Figs 4 and 5 , highly mobile endocytic vesicles around soma were excluded from analysis, since they unlikely reflect the local endocytosis related to proximal thinning (see description of Fig. 5 in Results). In these experiments, the proximal and distal dendrites correspond to those at average radial distance of less than ~100 μm and more than ~200 μm, respectively, relative to the soma. Photoactivation and FRAP experiments Photoactivation of PA-TagRFP was performed on an Olympus BX51WI upright microscope with the objective UPLFLN 40XO ( × 40 NA=1.3). The microscope and all the other components were controlled by Metamorph software. A digital-light-processing mirror array (MOSAIC, Photonics Instruments) was used to generate a spatial mask for delivering light for photoactivation. The spatial mask was generated at a region where the soma was located. A 405-nm ultraviolet laser (475 mW at max power, #LDCU8-220-3B/9079A, Power Technology) was used to photoactivate PA-TagRFP. Photoactivation was carried out within several minutes after C4da neurons had started spontaneous Ca 2+ transients. FRAP experiments were performed as follows: Ca 2+ imaging was performed first as described above. Just after neurons started Ca 2+ transients, the boundary between branch units and non-branch units was determined. Animals were then transferred to another confocal setup (Leica TCS SP8) and photobleaching was applied to a rectangle area covering the boundary. Immunostaining Immunostaining of Futsch . Animals raised at 33 °C from the onset of metamorphosis were dissected and fixed in 4% formaldehyde/PBS and stained with the mouse-anti-Futsch antibody (1:200; 22C10, Hybridoma Bank) at 6.5 h a.p.f. As secondary antibody, Cy3-conjugated anti-mouse antibody (1:200; Jackson Laboratory) was used. Z series images taken on a Leica TCS SP8 confocal microscope were projected onto a two-dimensional image file. Optical stimulation for accessing the dendritic excitability Optical stimulation and recording were performed by following our previous description, except that we induced the expression of the channelrhodopsin-2 (hChR2-EGFP) and RGECO1 by taking advantage of the Q-system [47] . The F1 generation of a cross between w; TrpA1-QF, QUAS-RGECO1 (on second chromosome) and w; +; TrpA1-QF, QUAS-ChR2-EGFP (on third chromosome) was used for the experiments. Analysis of the pruning phenotype Z series images taken on a Leica TCS SP8 confocal microscope were projected onto a two-dimensional image file. From the images, the length of dendrites was measured with Neuron J plugin in Image J software. Dendrites showing fragmentation or beading were excluded from the measurement. Because the results were not normally distributed, non-parametric statistics (that is, the Kruskal–Wallis test followed by a post hoc Steel–Dwass multiple comparison test) were applied. Induction of ca-beta mutant clones was performed as follows: embryos were collected for 2 h, allowed to develop for 3 h and then heat shocked for 30 min at 38 °C. The growing larvae were kept at 25 °C. Quantification of dendritic branch width Since the membrane-targeted fluorescent markers used in this study localize not only to the plasma membrane, but also to internal membranes (including endosomes), their fluorescent intensity could not reflect the dendritic branch width correctly. We therefore binalized the images to isolate labelled dendritic branches from the background and determine the outline of them, and used resulting binalized images for the quantification of dendritic branch width. Multiple rectangle regions of the same size were created along the binalized images of dendritic branches, and branch width was quantified as pixel count from each region. Analyses were performed by using Metamorph software. Statistics Statistical analyses were performed with SYSTAT 13 software (HULINKS, Tokyo, Japan) and R version 2.15.1 (The R Foundation for Statistical Computing). How to cite this article: Kanamori, T. et al. Local endocytosis triggers dendritic thinning and pruning in Drosophila sensory neurons. Nat. Commun. 6:6515 doi: 10.1038/ncomms7515 (2015).